Nanoscale sub-100 picosecond all-optical magnetization switching in GdFeCo microstructures Ultrafast magnetization reversal driven by femtosecond laser pulses has been shown to be a promising way to write information. Seeking to improve the recording density has raised intriguing fundamental questions about the feasibility of combining ultrafast temporal resolution with sub-wavelength spatial resolution for magnetic recording. Here we report on the experimental demonstration of nanoscale sub-100 ps all-optical magnetization switching, providing a path to sub-wavelength magnetic recording. Using computational methods, we reveal the feasibility of nanoscale magnetic switching even for an unfocused laser pulse. This effect is achieved by structuring the sample such that the laser pulse, via both refraction and interference, focuses onto a localized region of the structure, the position of which can be controlled by the structural design. Time-resolved photo-emission electron microscopy studies reveal that nanoscale magnetic switching employing such focusing can be pushed to the sub-100 ps regime. The ever-increasing demands for faster and denser magnetic recording has been continuously fueling the search for ways to control magnetization in a medium by means other than magnetic fields. Several approaches based on excitation by intense Teraherz pulses [1] , [2] , [3] , electric fields [4] , [5] , [6] , spin-polarized currents [7] , [8] , [9] , [10] or strain pulses [11] , [12] are possible candidates for the manipulation of magnetism at time scales shorter than 100 ps. In particular, femtosecond visible laser pulses have been shown to offer extensive control of demagnetization [13] and magnetic reversal [14] for a wide range of materials, including insulators and metals for both ferro- and antiferro-magnetic order [15] . Of particular interest to magnetic recording applications is the magnetization reversal induced by a single femtosecond laser pulse, which was first reported in GdFeCo ferrimagnetic amorphous alloys [14] . Although a detailed microscopic understanding of this all-optical switching (AOS) phenomena is still lacking, different models have been proposed. The originally proposed mechanism based on the non-thermal inverse Faraday effect and helicity-dependent switching is still being discussed [14] , [16] , [17] , [18] . Another model relies on the formation of a transient ferromagnetic-like state between the Fe and Gd sub-lattices [19] . A total angular momentum conserving exchange of spin moments between the two magnetic sub-lattices has been suggested to explain this ultrafast counter-intuitive magnetization dynamics [20] , [21] . Such magnetization dynamics can be triggered whenever a heat load brings the magnetic sub-lattices out of equilibrium and does not require the presence of a magnetic field nor light of a particular polarization [22] . Finally, the role of laser-induced super-diffusive spin currents in alloys is being discussed [23] , [24] . Besides the obvious attractiveness of recording information with ultrashort femtosecond excitations, AOS displays numerous interesting features in view of potential applications. First of all, the range of systems where AOS has been observed is continuously increasing. Initially reported in GdFe-based ferrimagnetic alloys, it has then been observed in other rare earth-transition metal alloys [25] and multilayers [26] , as well as rare-earth free-based ferri- [16] , [27] and ferromagnetic multi-layers [17] , making AOS a rather general phenomena. Second, AOS is an energy-efficient process, with <10 fJ of energy necessary to reverse a 20 nm × 20 nm magnetic domain in GdFeCo [28] . Third, it is possible to write the desired ‘up’ or ‘down’ magnetic domain orientation by selecting the appropriate left- or right-handed circularly polarized laser pulse, taking advantage of the magnetic circular dichroism of the recording media in combination with the threshold behaviour of AOS [29] . Finally, laser pulses can be focused with plasmonic antennae to spot sizes of a few tens of nanometres [30] , [31] , [32] , [33] . However, whether nanoscale sub-100 ps all-optical magnetization switching is feasible remains to be tested. Here we report the experimental demonstration of nanoscale and sub-100 ps all-optical magnetization switching employing linearly polarized laser pulses. Using finite-difference time-domain (FDTD) methods to simulate the laser absorption profile within the magnetic structure, we reveal the feasibility of nanoscale magnetic switching even for the case of an unfocused incoming laser pulse. This effect originates from the laser pulse coupling and propagating within the magnetic structure where it experiences a complex combination of refraction and interference that leads to its focusing onto a localized region of the structure. This effect is found to persist down to structural sizes of 5 nm × 5 nm. Time-resolved studies with the help of photo-emission electron microscopy (PEEM), using X-ray magnetic circular dichroism (XMCD) as a contrast mechanism in magnetic structures down to 1 μm × 1 μm, clearly reveal that the sub-wavelength AOS employing the focusing properties of the structure can be pushed into sub-100 ps regime. Simulated light absorption in GdFeCo structures To demonstrate sub-wavelength all-optical magnetization switching, one would think of employing near-field plasmonic antennae to focus the laser pulse down to a few tens of nanometres [30] , [31] , [32] , [33] . However, the coupling of the laser pulse with small structures is a non-trivial problem. We thus investigated the electromagnetic wave propagation of a femtosecond laser pulse inside a magnetic structure using FDTD simulations. For the modelling, we have chosen a realistic GdFeCo multilayer structure, which is known to display all-optical magnetization switching (AOS), that is, the ability to reverse permanently its magnetization on the sole influence of a femtosecond laser pulse [14] . The simulations of the light absorption profiles A were performed for different structural sizes ranging from 5 μm × 5 μm down to 5 nm × 5 nm. The results are shown in Fig. 1 . Although the 16° grazing incidence geometry was kept constant in these simulations, the in-plane incoming laser direction defined as the angle between the in-plane laser wave vector k and one edge of the structure was varied. The results for 0° and 45° are shown in Fig. 1a–f and g–l , respectively. The first striking feature is that even though the incoming laser pulse is a plane wave with a 800-nm wavelength, that is, orders of magnitude larger than the smallest simulated structure, the light absorption A inside the structure is inhomogeneous down to the 5 nm × 5 nm structure in Fig. 1f,l . These absorption profiles also depend strongly on the incoming laser direction with respect to the structure edge, as can be seen by a direct comparison between Fig. 1a–f and g–l . In particular, an interesting case occurs at 45° where the absorbed laser energy is mostly confined within a quarter of the structure, as shown in Fig. 1i in the top right corner, as well as in Fig. 1j in the opposite bottom left corner. Moreover, these absorption profile inhomogeneities are rather strong, displaying a ratio of ~2 between the highest and lowest absorption regions inside the structures down to the 20 nm × 20 nm structure shown in Fig. 1d,j . This ratio reduces to 1.5 for the 10 nm × 10 nm structure shown in Fig. 1e,k and to 1.1 for the 5 nm × 5 nm structure shown in Fig. 1f,l . Furthermore, the total absorbed energy increases by a factor of 2 from the largest to the smallest structures, making the smaller structures more absorbing and thus more energy efficient as previously reported [28] . 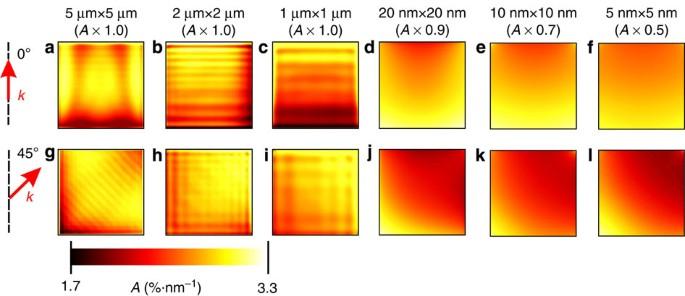Figure 1: Simulated light absorption as a function of structure size and incoming laser direction. FDTD-simulated light absorptionAinside structures of different sizes ranging from 5 μm × 5 μm (a,g) down to 5 nm × 5 nm (f,l). The simulations are shown for two different incoming laser directions with respect to the structure edge as shown in the inset by the in-plane light wave vectorkat 0° for (a–f) and at 45° for (g–l). In both cases, the laser light impinges with a 16° grazing incidence. The absorption profilesAhave been scaled by the factor indicated in the parentheses such that they all fall into the same range. Figure 1: Simulated light absorption as a function of structure size and incoming laser direction. FDTD-simulated light absorption A inside structures of different sizes ranging from 5 μm × 5 μm ( a , g ) down to 5 nm × 5 nm ( f , l ). The simulations are shown for two different incoming laser directions with respect to the structure edge as shown in the inset by the in-plane light wave vector k at 0° for ( a – f ) and at 45° for ( g – l ). In both cases, the laser light impinges with a 16° grazing incidence. The absorption profiles A have been scaled by the factor indicated in the parentheses such that they all fall into the same range. Full size image These focusing and coupling efficiency effects are created by the structure’s boundaries and the interference between the waves propagating and absorbing within the sample. It must be noted that these effects are not only present at 16° grazing incidence as shown here but also at normal incidence as previously shown by simulation [28] . The grazing incidence geometry offers an additional degree of freedom such that depending on the orientation of the boundary with respect to the propagation wave vector of the light pulse, different continuity relations take place, resulting in different Fresnel coefficients [34] . This leads, for example, to the intense side lobes seen in the 5 μm × 5 μm structure at 0° incoming azimuthal direction shown in Fig. 1a . Refraction, reflection and interference of these waves occurring within the structure, which are best seen in the 45° incoming direction cases shown in Fig. 1h , create strong intensity variations inside the structure. Strong optical absorption of light leads to the formation of these features on the length scale of a few nanometres. These simulations demonstrate that in the case of an incoming laser pulse at grazing incidence, it is possible to focus the laser pulse by the structural geometry such that the absorption is confined into parts of the structure, which are well below the far field diffraction limit. These results pose the question as to whether or not such systems can be employed to all-optically switch a nanoscale region of a magnetic structure. The answer to this question will now be addressed. Time-resolved magnetization dynamics in GdFeCo structure AOS occurs via the energy absorbed from the laser pulse [22] and displays a switching threshold behaviour [29] . This means that below a certain laser fluence, or more precisely, below a certain absorbed energy density, only partial demagnetization occurs and the sample magnetization recovers to its initial state. Above this threshold fluence, deterministic magnetization switching occurs. At even higher fluence, the magnetization switching disappears and randomly oriented domains are created with no relation to the initial state. Thus, by investigating the spatially resolved magnetization state in GdFeCo structures after laser pulse excitation, as a function of the laser fluence, it is possible to study the passive focusing experienced by the laser pulse interacting with the structure and to determine whether partial magnetization switching of the structure is feasible. However, due to the low coercivity of the GdFeCo alloys, the switched domains are likely to reorganize after switching on the relevant length scale, which here is a few hundred of nanometres. It is therefore necessary for the sample investigated to probe the magnetization shortly after the laser pulse. For this, time-resolved XMCD PEEM imaging was employed, which offers magnetic domain imaging with 70 ps time resolution and ~200 nm spatial resolution in time-resolved mode. By fixing the time delay t between the laser pump and the X-ray probe, the spatially resolved intermediate magnetization state inside a structure at that specific time delay can be recorded. The time-resolved XMCD images for a 5 μm × 5 μm square microstructure at t =400 ps after the laser pulse as a function of the incoming laser fluence, , are shown in Fig. 2a for an incoming laser direction along the structure edge, and in Fig. 2d for an incoming laser direction of 45° from the structure edge. It is important to note that at this relatively long time delay of a few hundred picoseconds, both the Gd and the FeCo sub-lattice magnetization are again in equilibrium with each other, such that measuring only one sub-lattice is enough to characterize the sample magnetization [19] . On the other hand, this time scale is short enough to probe the transient longitudinal magnetization dynamics occurring, in particular whether partial, total demagnetization or magnetization switching has taken place. The initial state of this microstructure is mono-domain due to a static out-of-plane magnetic field of 50 mT applied along its magnetic easy axis, which displays itself as a homogeneous white XMCD contrast. For the low fluence case of shown in Fig. 2a , one can see that the contrast is no longer uniform, and that some partial demagnetization has occurred at the centre of the structure. As the fluence is increased, the contrast displayed by each area within the microstructure changes from white to black, and further from black to grey. To understand what these contrast changes correspond to, it is necessary to look at the magnetization dynamics of each area. 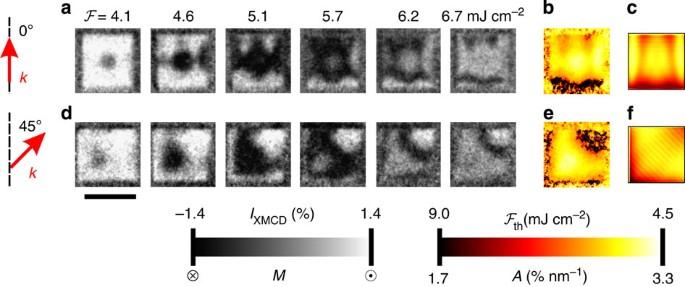Figure 2: Experimentally observed magnetization switching patterns for a 5 μm × 5 μm GdFeCo structure. (a) Time-resolved PEEM images using XMCD as a magnetic contrast mechanism as a function of the incoming laser fluenceand for an incoming laser direction with respect to the structure edge of 0° as indicated in the inset by the laser in-plane wave vectork. All images are recorded at a fixed time delay oft=400 ps after the laser pulse. (d) Same as before but for a 45° incoming laser direction. (b,e) The extracted spatially resolved fluence switching thresholdfor the 0° and the 45° incoming laser direction, respectively. (c,f) The FDTD-simulated light absorptionAinside the 5 μm × 5 μm structures for the 0° and the 45° incoming laser direction, respectively. The grey scale indicates the relation between the XMCD image contrastIXMCDand the out-of-plane magnetization componentMbeing inward⊗or outward. Scale bar, 5 μm. Figure 2: Experimentally observed magnetization switching patterns for a 5 μm × 5 μm GdFeCo structure. ( a ) Time-resolved PEEM images using XMCD as a magnetic contrast mechanism as a function of the incoming laser fluence and for an incoming laser direction with respect to the structure edge of 0° as indicated in the inset by the laser in-plane wave vector k . All images are recorded at a fixed time delay of t =400 ps after the laser pulse. ( d ) Same as before but for a 45° incoming laser direction. ( b , e ) The extracted spatially resolved fluence switching threshold for the 0° and the 45° incoming laser direction, respectively. ( c , f ) The FDTD-simulated light absorption A inside the 5 μm × 5 μm structures for the 0° and the 45° incoming laser direction, respectively. The grey scale indicates the relation between the XMCD image contrast I XMCD and the out-of-plane magnetization component M being inward ⊗ or outward . Scale bar, 5 μm. Full size image The spatially resolved magnetization dynamics inside a 5 μm × 5 μm microstructure recorded with time-resolved XMCD PEEM are shown for two different incoming laser fluences of in Fig. 3a and of in Fig. 3c . In both cases, a 16° grazing incidence and a 0° incoming laser direction with respect to the structure edge was used, as indicated by the inset in Fig. 3b,d . Three different regions of interest (ROI) have been defined, and for each the time-dependent magnetic contrast is extracted. The first ROI in red at the centre of the structure corresponds to the region in Fig. 2a that changes contrast at the lowest fluence. The second ROI in green corresponds to an intermediate case and the third ROI in blue corresponds to a region that begins to change contrast at the highest fluence. For each of these three differents ROI, the averaged XMCD contrast is extracted and displayed as a function of the time delay t in Fig. 3b,d , for the low and high fluence, respectively. In case of the low incoming fluence shown in Fig. 3b , only the red ROI shows a magnetization switching, while both other regions show only a partial demagnetization. This means that the contrast change from white to black in Fig. 2a corresponds to the onset of AOS as the fluence is increased. Increasing the fluence further, the magnetization dynamics of each region drastically changes, as seen in Fig. 3d . Now, only the green ROI switches, whereas the red ROI (which was switching at lower fluence) now only displays a demagnetization followed by a recovery to the initial state on cooling under the action of the applied out-of-plane magnetic field. This means that the contrast change from black to grey observed in Fig. 2a corresponds to the loss of deterministic switching when the fluence is increased too far. This is essentially the known phase diagram of the fluence dependence of AOS, with its threshold behaviour [29] . 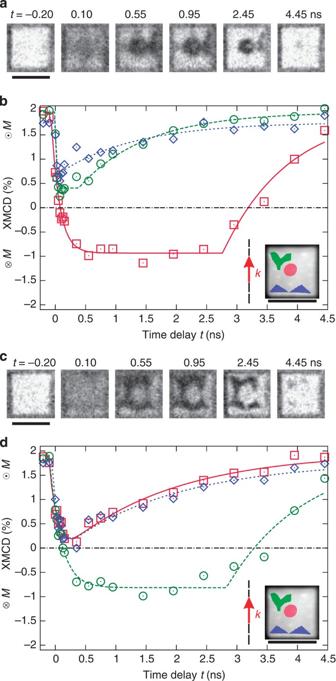Figure 3: Magnetization dynamics inside a 5 μm × 5 μm structure. (a) Time-resolved PEEM images using XMCD as a magnetic contrast mechanism recorded at a given time delaytafter the laser pulse and (b) extracted XMCD contrast as a function of the time delaytfor three different ROI, defined in the inset image by the coloured area superimposed on the non-dichroic X-ray absorption of the structure. The red ROI corresponds to the centre of the structure, which switches at the lowest fluence; the green region to a part of the top left corner, which switches at intermediate fluence; and the blue region to the bottom part of the structure, which switches at the highest fluence. The points are the measured data, whereas the lines are guides to the eye. The 0° incoming laser direction with respect to the structure edge is indicated in the inset by the laser in-plane wave vectork. The corresponding inward⊗or outwardout-of-plane magnetization componentMare indicated on the XMCD axis. The incoming laser fluence was. (c,d) The same for an incoming laser fluence of. Scale bars, 5 μm. Figure 3: Magnetization dynamics inside a 5 μm × 5 μm structure. ( a ) Time-resolved PEEM images using XMCD as a magnetic contrast mechanism recorded at a given time delay t after the laser pulse and ( b ) extracted XMCD contrast as a function of the time delay t for three different ROI, defined in the inset image by the coloured area superimposed on the non-dichroic X-ray absorption of the structure. The red ROI corresponds to the centre of the structure, which switches at the lowest fluence; the green region to a part of the top left corner, which switches at intermediate fluence; and the blue region to the bottom part of the structure, which switches at the highest fluence. The points are the measured data, whereas the lines are guides to the eye. The 0° incoming laser direction with respect to the structure edge is indicated in the inset by the laser in-plane wave vector k . The corresponding inward ⊗ or outward out-of-plane magnetization component M are indicated on the XMCD axis. The incoming laser fluence was . ( c , d ) The same for an incoming laser fluence of . Scale bars, 5 μm. Full size image The same experiments were repeated in 2 μm × 2 μm and 1 μm × 1 μm structures, for a fluence of and an incoming laser direction of 45° with respect to the structure edge. The recorded magnetization dynamics is shown in Fig. 4a . In these structures, the switching patterns are notably different from the previous case of the larger 5 μm × 5 μm structures shown in Fig. 3a due to the different structure size and the different incoming laser direction as shown in Fig. 1 . In this case, the ROI are defined as the top right corner in blue and red for the 2 μm × 2 μm and 1 μm × 1 μm structures, respectively, and the bottom left corner in yellow and green for the 2 μm × 2 μm and 1 μm × 1 μm structures, respectively. In the extracted magnetization dynamics of each region shown in Fig. 4b , we observe that both the 2 μm × 2 μm and 1 μm × 1 μm structures simultaneously host a region displaying AOS in blue and red, and a region displaying demagnetization followed by a quick recovery to the initial state in yellow and green. In the 1 μm × 1 μm structure in particular, the red region showing AOS is ~300 nm wide, which is notably smaller than the free space diffraction limit at this wavelength. This can be understood by considering that the wavelength of the light propagating inside the GdFeCo layer is approximately four times smaller than in vacuum due to the GdFeCo refractive index. Experiments performed on smaller structures were limited by the photo-emitted electron count statistics and the instrument spatial resolution in this time-resolved mode. 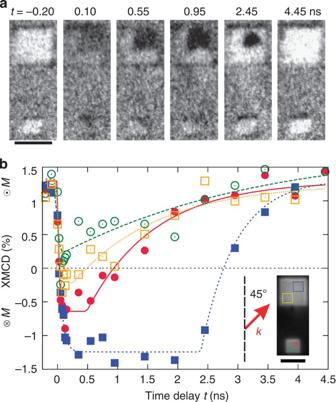Figure 4: Magnetization dynamics inside a 2 μm × 2 μm and 1 μm × 1 μm structures. (a) Time-resolved PEEM images using XMCD as a magnetic contrast mechanism recorded at a given time delaytafter the laser pulse and (b) extracted XMCD contrast as a function of the time delaytfor four different ROI, defined in the inset image by the colured area superimposed on the non-dichroic X-ray absorption of the structure. The blue and yellow ROI corresponds to the top right and bottom left corner region of the 2 μm × 2 μm structure, respectively. The red and green ROI corresponds to the top right and bottom left corner region of the 1 μm × 1 μm structure, respectively. In both cases, the top right ROI shows switching, whereas the bottom left shows only demagnetization. The points are the measured data, whereas the lines are guides to the eye. The 45° incoming laser direction with respect to the structure edge is indicated in the inset by the laser in-plane wave vectork. The corresponding inward⊗or outwardout-of-plane magnetization componentMare indicated on the XMCD axis. The incoming laser fluence was. Scale bars, 2 μm. Figure 4: Magnetization dynamics inside a 2 μm × 2 μm and 1 μm × 1 μm structures. ( a ) Time-resolved PEEM images using XMCD as a magnetic contrast mechanism recorded at a given time delay t after the laser pulse and ( b ) extracted XMCD contrast as a function of the time delay t for four different ROI, defined in the inset image by the colured area superimposed on the non-dichroic X-ray absorption of the structure. The blue and yellow ROI corresponds to the top right and bottom left corner region of the 2 μm × 2 μm structure, respectively. The red and green ROI corresponds to the top right and bottom left corner region of the 1 μm × 1 μm structure, respectively. In both cases, the top right ROI shows switching, whereas the bottom left shows only demagnetization. The points are the measured data, whereas the lines are guides to the eye. The 45° incoming laser direction with respect to the structure edge is indicated in the inset by the laser in-plane wave vector k . The corresponding inward ⊗ or outward out-of-plane magnetization component M are indicated on the XMCD axis. The incoming laser fluence was . Scale bars, 2 μm. Full size image From the FDTD simulations shown in Fig. 1 , it is seen that the structural orientation and size produce a complex combination of refraction and interference such that the laser energy is focused onto only part of the structure. Thus, the designing of the structural geometry allows focusing of the laser pulse and these effects persist to structural sizes as small as 5 nm × 5 nm. Comparing the absorption profile A obtained from the FDTD simulations ( Fig. 2c,f for a 0° and 45° incoming laser direction, respectively) with the fluence threshold patterns obtained from the experiments ( Fig. 2b,e , respectively), a direct relation between the two is revealed. Moreover, the fact that the resulting pattern completely changes with the incoming laser direction between Fig. 2b,e rules out an intrinsic inhomogeneous switching threshold due to, for example, chemical inhomogeneities in the structure composition whose effects have been seen in other studies [24] . Thus, it is not the fluence threshold , which varies inside the structure, but rather the light absorption A , as shown in Fig. 1 , even though the laser spot size of 30 μm × 105 μm is much larger than the structure itself. Very good qualitative agreement is obtained, as a region with a low corresponds to a region with high absorption and vice versa. The agreement is even reasonably quantitative as the ratio between the high and low fluence threshold is approximately a factor of 2, in accordance with the ratio between high and low absorption. Furthermore, these different absorption patterns directly translate to correspondingly different magnetization dynamics, as shown in Fig. 3a,c and in Fig. 4a . In particular, from the magnetization dynamics of the 1 μm × 1 μm structure shown in Fig. 4b , it is seen that a 300-nm wide magnetic domain is transiently reversed, demonstrating spatially selective AOS. It is to be noted that the whole structure relaxes to the initial state due to the applied out-of-plane magnetic field. Although this is a requirement for the present stroboscopic pump–probe experiments in GdFeCo samples, it is not a requirement for the observation of spatially selective switching. In the case of a rare earth-transition metal alloy with a much higher magnetic anisotropy, for example TbFeCo, the reversed pattern induced by the laser pulse inside the microstructure would be stable at smaller sizes [35] . Thus, employing the focusing properties of the structure itself, an inhomogeneously absorbed laser energy is obtained at the nanoscale, which in turn triggers inhomogeneous magnetization dynamics. This allows for a selective all-optical magnetization switching inside the microstructure, even though the incoming laser pulse is homogeneously illuminating the structure. These results open novel opportunities for very-high-density data storage media, for example, by either recording several bits of information in a single magnetic structure or by improving the coupling efficiency between the laser pulse and the magnetic structure. Finite-difference time-domain simulations Electromagnetic wave propagation within the structures was simulated with a commercial-grade simulator based on the FDTD method [36] . Various micro- and nanostructures with squared and circular shape were simulated. They consisted of multilayered structures ranging in area from 5 μm × 5 μm down to 5 nm × 5 nm. A variable three-dimensional discretization mesh was used as a function of the pattern size, with volume elements ranging from 15 nm × 15 nm × 1 nm for the largest structure down to 0.1 nm × 0.1 nm × 1 nm for the smallest. We considered a plane wave illumination at a wavelength λ =800 nm, linearly p -polarized, impinging on the sample with a grazing incidence angle of 16° (74° from the normal). These settings are chosen to correspond to the experimental conditions, where a Gaussian profile beam is used as illumination having a full width at half maximum (FWHM) much larger than the structural size. We also used a Gaussian profile with dimensions comparable to the experimental ones, without observing substantial differences with the simulations performed with plane-wave illumination. The structures all sit on a silicon substrate with a complex index of refraction ñ Si =n+ i k=3.692+0.0065 i (ref. 37 ), while the upper half space is vacuum. The structures are composed of several layers, namely, starting from the bottom one, AlTi(10 nm)/Si 3 N 4 (5 nm)/GdFeCo(20 nm)/Si 3 N 4 (3 nm). The refractive indexes of the layers are ñ AlTi =2.81+5.89 i , calculated as an average of ñ Al and ñ Ti from ref. 37 , (ref. 37 ) and ñ GdFeCo =3.7+3.856 i (ref. 32 ). The light absorption , where E is the light electric field, is mapped at the centre of the GdFeCo layer. A good convergence of the simulations was obtained with variable time steps <0.1 fs and a total simulation time of ~100 fs, while the Fourier-transform-limited laser pulse was ~10 fs long. Sample preparation and microstructuring The sample consisted of a multilayer thin film of composition AlTi(10 nm)/Si 3 N 4 (5 nm)/Gd 24 Fe 66.5 Co 9.5 (20 nm)/Si 3 N 4 (3 nm) grown by magnetron sputtering on a silicon substrate and are essentially the same as in ref. 38 . The structuring of these samples in squares and discs with sizes ranging from 5 μm × 5 μm down to 1 μm × 1 μm has been realized via electron beam lithography in combination with a lift-off process, in which a polymethylmethacrylate resist is first patterned with an electron beam writer on a Si substrate. This pattern is then transferred via lift-off after deposition by magnetron sputtering of the magnetic multilayer AlTi(10 nm)/Si 3 N 4 (5 nm)/Gd 24 Fe 66.5 Co 9.5 (20 nm)/Si 3 N 4 (3 nm), resulting in isolated magnetic structures [39] . Unstructured areas of several 100 μm, quasi-continuous films and arrays of squares and disks down to 100 nm were fabricated onto the same sample. In the manuscript, we focus only on the 5 μm × 5 μm, 2 μm × 2 μm and 1 μm × 1 μm squares, as simulations for larger structures are too time consuming and the signal-to-noise ratio for smaller structures is too small. Time-resolved magnetization dynamics measurements Spatially resolved images of the magnetic domain states in these microstructures were obtained with the Elmitec PEEM at the surface/interface: microscopy beamline [40] at the Swiss Light Source using the XMCD effect at the Fe L 3 -edge at 708 eV as a magnetic contrast mechanism. An XMCD asymmetry image is obtained by taking two total electron yield images measured with opposite X-ray helicities at resonant energies. The resulting contrast is proportional to the scalar product of the local magnetization and the incoming X-ray wave vectors [41] , that is, the more parallel the magnetization is to the X-ray wave vector, the brighter the contrast. Time-resolved measurements were performed by taking advantage of the pulsed nature of the X-rays produced by the Swiss Light Source synchrotron via the gating of the detection in synchronization to an isolated electron bucket present in the gap of the filling pattern of the storage ring. This scheme, presented in details in ref. 42 , allows stroboscopic pump–probe imaging of the sample with a time resolution determined by the 70 ps FWHM X-ray pulse length. To perform stroboscopic measurements, the magnetic state of the sample is recovered after each pump event, thanks to a permanent magnet mounted directly underneath the sample and saturating it with an out-of-plane magnetic field of 50 mT. The laser used for the pump is produced by an XL-500 oscillator from Femtolasers Produktions GmbH and characterized by a τ =50 fs laser pulse length at λ =800 nm wavelength, with 500 nJ per pulse at a 5.2 MHz repetition rate. The laser is then focused on the sample at a grazing incidence of 16° to a FWHM spot size of 30 μm vertically and 105 μm horizontally. Finally, the sample can be azimuthally rotated in situ to perform experiments at different incoming laser directions. How to cite this article : Le Guyader, L. et al. Nanoscale sub-100 picosecond all-optical magnetization switching in GdFeCo microstructures. Nat. Commun. 6:5839 doi: 10.1038/ncomms6839 (2015).